Division of labour between Myc and G1 cyclins in cell cycle commitment and pace control A body of evidence has shown that the control of E2F transcription factor activity is critical for determining cell cycle entry and cell proliferation. However, an understanding of the precise determinants of this control, including the role of other cell-cycle regulatory activities, has not been clearly defined. Here, recognizing that the contributions of individual regulatory components could be masked by heterogeneity in populations of cells, we model the potential roles of individual components together with the use of an integrated system to follow E2F dynamics at the single-cell level and in real time. These analyses reveal that crossing a threshold amplitude of E2F accumulation determines cell cycle commitment. Importantly, we find that Myc is critical in modulating the amplitude, whereas cyclin D/E activities have little effect on amplitude but do contribute to the modulation of duration of E2F activation, thereby affecting the pace of cell cycle progression. E2F transcriptional factors are a family of proteins that bind to overlapping sets of target promoters, regulating cell cycle progression and cell-fate decisions [1] , [2] , [3] , [4] , [5] , [6] . Enforced E2F1 expression can induce quiescent cells to enter S phase, and genetic loss of all activator E2Fs (E2F1-3) completely abolishes the ability of normal fibroblasts to enter S phase [7] , [8] . Substantial evidence supports the view that the Rb/E2F network ochestrates the precise regulation of E2F activation [2] , [4] , [9] , [10] , [11] ( Fig. 1 ). The canonical view is that mitogen-driven expression of D-type cyclins and activation of their partners cyclin-dependent kinase (CDK) 4/6 initialize the phosphorylation of Rb, releasing existing E2F protein from Rb sequestration [12] . Free E2F can then transcribe Cyclin E, which together with CDK2, hyper-phosphorylates Rb, resulting in full activation of E2F [13] . The potent oncogene, Myc, dramatically affects E2F activity, presumably through modulating G1 cyclins expression as well as cyclin-dependent kinase (CDK) activities [14] . However, restoration of Cyclin D level, despite succeeding in restoring the kinetics of Rb phosphorylation to normal, fails to rescue slow-growth phenotypes in c-Myc-deficient cells [15] , [16] . Moreover, it was recently showed that Myc is also required for allowing the interaction of the E2F protein with the E2F gene promoters [17] , [18] , suggesting a direct and Rb-independent regulatory role of Myc on E2F activation through interfering with E2F auto-regulation. In addition, several target genes of E2F, such as Cyclin A and Skp2, contribute to negative feedback loops and affect E2F activity through direct regulation of its transcriptional activity or protein degradation [19] , [20] . 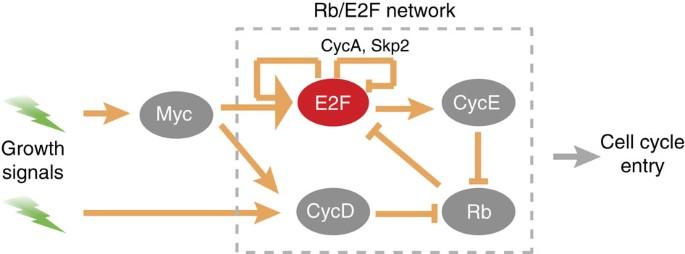Figure 1: A diagram of Myc-regulated Rb/E2F network. The canonical Rb/E2F network is highlighted with a dashed rectangle. CycD and CycE represent Cyclin D/CDK4/6 complex and Cyclin E/CDK2 complex, respectively. Figure 1: A diagram of Myc-regulated Rb/E2F network. The canonical Rb/E2F network is highlighted with a dashed rectangle. CycD and CycE represent Cyclin D/CDK4/6 complex and Cyclin E/CDK2 complex, respectively. Full size image It has been generally accepted that the commitment into cell cycle is determined by E2F activation because of G1 cyclin/CDK complexe-mediated Rb phosphorylation. However, it appears difficult to reconcile this view with the observation that major phosphorylation of Rb occurs after the restriction point [21] , [22] ; other events may be more critical for the initial E2F activation. Conventional approaches based on population analysis cannot adequately address this question, in light of extensive heterogeneity in gene expression among cells that can mask or obfuscate the contributions from different regulatory elements [23] , [24] . Single-cell analysis provides the opportunity to follow the dynamics of signalling molecules that reflect how an individual cell encodes and decodes information that result in a particular cellular outcome [24] , [25] , [26] , [27] , [28] , [29] , [30] . To this end, we used time-lapse fluorescence microscopy to follow E2F1 temporal dynamics in single cells. Guided by mathematical modelling, we set out to address several specific questions. In particular, do E2F dynamics determine the commitment to cell cycle entry in individual cells? If so, what aspects of E2F temporal dynamics are the major determinants of cell cycle entry? How do Myc and G1 cyclins affect different aspects of E2F temporal dynamics? How do their effects manifest themselves in the ability of a single cell to enter and pace the cell cycle? In contrast to the canonical view, our results reveal that Myc and G1 cyclins contribute to distinct aspects of the E2F temporal dynamics, despite their apparently overlapping roles. In particular, Myc primarily sets the maximum E2F level, which in turn determines commitment to cell cycle entry. G1 cyclins, however, control the timing for reaching the maximum level and thus the pace of cell cycle progression. We find that these distinctive modes of control over the E2F temporal dynamics are an intrinsic dynamic property of the core Rb/E2F network. On one hand, our results elucidate the different roles that Myc and G1 cyclins play in controlling cell cycle entry and progression. On the other hand, this ‘division of labour’ represents a novel, perhaps general, strategy to integrate different signals (Myc versus G1 cyclins) through a common ‘signal carrier’ (E2F). Quantification of E2F dynamics in single cells To measure E2F1 transcriptional dynamics in single cells, we re-engineered the reporter construct from Yao et al. [4] to generate a brighter fluorescent signal that is largely localized to the nucleus ( Fig. 2a ). The improvements facilitated segmentation and signal extraction in individual cells, as nuclei are well separated from each other in the field of observation. Individual cell clones (REF52-hE2F1p::4NLS-d4Venus) expressing the reporter construct were isolated and used for experimental validation. Consistent with our expectations, the majority of the Venus fluorescence signal in independent clones was restricted to the nucleus, with a small amount of the signal localized around the nucleus ( Fig. 2b ). We confirmed that the reporter recapitulated E2F1 dynamics at the population level by comparing the individual trajectories and endogenous E2F1 mRNA expression over time ( Supplementary Fig. 1a ). Furthermore, we found that the accumulation of Venus and endogenous E2F1 proteins were also concordant, although minor differences can be seen, particularly in later time points ( Supplementary Fig. 1b ). Altogether, the dynamic expression of the reporter correlated with endogenous E2F1 expression throughout the time course of the experiment. 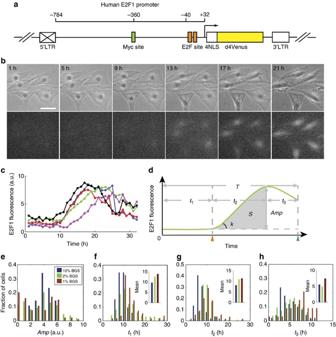Figure 2: Quantification of E2F dynamics in single cells. (a) hE2F1p::4NLS-d4Venus reporter construct. Box with cross indicates that 5′ long terminal repeat (LTR) is inactivated after viral integration. (b) Time-lapse microscopy images of REF52 rat fibroblasts expressing hE2F1p::4NLS-d4Venus reporter released from serum starvation by adding 10% bovine growth serum (BGS). Upper panel, phase channel; low panel, Venus channel. Scale bar, 50 μm. (c) E2F1 dynamics trajectories of the five individual cells shown inb. Time-series raw data (sampled per hour) were smoothened in a 3-h time window. (d) Characterization of E2F1 dynamics trajectory in divided (green) cells with defined metrics:t1, initial delay;t2, activation time;t3, post-activation time;Amp, amplitude;S(shadow area), total E2F1 work during activation time;k, slope;T, the entire cell cycle length. Orange triangle indicates E2F1 signal upturn time point and the blue one indicates cell division time point. (e) Histogram shows the distribution ofAmpat different serum levels. (f–h) Histograms show distributions oft1,t2andt3(in divided cells) at different serum levels. The mean values were compared among different serum concentrations and plotted as insets. Figure 2: Quantification of E2F dynamics in single cells. ( a ) hE2F1p::4NLS-d4Venus reporter construct. Box with cross indicates that 5′ long terminal repeat (LTR) is inactivated after viral integration. ( b ) Time-lapse microscopy images of REF52 rat fibroblasts expressing hE2F1p::4NLS-d4Venus reporter released from serum starvation by adding 10% bovine growth serum (BGS). Upper panel, phase channel; low panel, Venus channel. Scale bar, 50 μm. ( c ) E2F1 dynamics trajectories of the five individual cells shown in b . Time-series raw data (sampled per hour) were smoothened in a 3-h time window. ( d ) Characterization of E2F1 dynamics trajectory in divided (green) cells with defined metrics: t 1 , initial delay; t 2 , activation time; t 3 , post-activation time; Amp , amplitude; S (shadow area), total E2F1 work during activation time; k , slope; T , the entire cell cycle length. Orange triangle indicates E2F1 signal upturn time point and the blue one indicates cell division time point. ( e ) Histogram shows the distribution of Amp at different serum levels. ( f – h ) Histograms show distributions of t 1 , t 2 and t 3 (in divided cells) at different serum levels. The mean values were compared among different serum concentrations and plotted as insets. Full size image We next used this proxy system to examine the real-time dynamics of E2F in single REF52 rat fibroblasts held in G0 through serum starvation and released into the cell cycle by serum stimulation. For each time point, we quantified the level of fluorescence in individual cells, which could be accurately measured up to early M phase, when the nuclear membrane starts to fall apart ( Fig. 2b , Supplementary Movies 1 and 2 ). The temporal E2F dynamics in individual cells were highly variable ( Fig. 2c ), but exhibited a consistent pattern: after an initial delay, the E2F1 signal increased from a basal level to a maximum value and then slowly decreased ( Fig. 2d ). Moreover, the same overall pattern was observed in single cells isolated from other clones transduced independently with our reporter gene. We then defined a set of metrics to quantify the observed E2F dynamics ( Fig. 2d ). These include maximum amplitude ( Amp ), initial delay ( t 1 ), activation time ( t 2 ) and post-activation time ( t 3 , for cells that undergo division only). Amp and t 2 can be combined to define two additional metrics—the slope ( k = Amp / t 2 ) and the area under the curve ( S = Amp × t 2 /2); k corresponds to the rate increase, which reflects the strength of positive feedback loop in the regulation, whereas S correlates with the total transcription work of the network directed at the E2F1 promoter ( Fig. 2d ). See Fig. 2d legend for additional definitions. To evaluate these metrics, we measured E2F1 temporal dynamics in ~100 individual cells for each level of serum activation and calculated their values for each cell. Values of the four metrics (as shown for Amp , t 1 , t 2 and t 3 ) were highly variable among individual cells ( Fig. 2e–h ) because of stochastic gene expression. Notably, Amp exhibited bimodal distribution (ON/OFF) at an intermediate serum concentration ( Fig. 2e ), consistent with the bistability of the Rb/E2F switch [4] . Moreover, decreasing serum concentration led to significant change in the distribution of Amp but moderate increase of average values of t 1 , t 2 and t 3 ( Fig. 2e–h ). Pairwise correlation analyses revealed a weak correlation between Amp and t 2 , and no significant correlations between other pairs, suggesting little dependence among these metrics ( Supplementary Fig. 1c ). Amp as the predictor of commitment and division We next examined the extent by which the metrics defined above could predict cell-cycle entry commitment and proliferation ( Fig. 3a ). To this end, we combined measurements of single-cell E2F dynamics with measurement of 5-ethynyl-2′-deoxyuridine (EdU) incorporation into newly synthesized DNA, a surrogate for determining cell cycle entry ( Fig. 3b and c ). We found that Amp is a reliable predictor of commitment. Specifically, plotting EdU signals against Amp values for ~100 cells revealed two distinct groups of cells: cells with high EdU incorporation had an Amp value above a threshold ( Amp th ), whereas cells with no EdU labelling showed a value of Amp below it ( Fig. 3d ). Two Amp -related metrics— k and S —were also informative, albeit less accurate at predicting cell cycle entry ( Supplementary Fig. 2a and b ). The other metrics ( t 1 and t 2 ) were much less reliable predictors ( Supplementary Fig. 2c and d ). 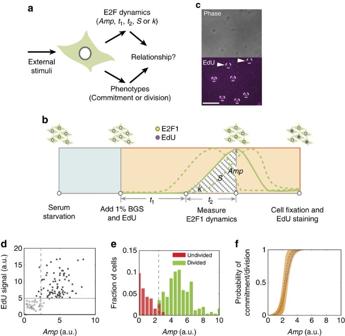Figure 3:Ampas the predictor of commitment and division. (a) Linking E2F dynamics to phenotypes in single cells. (b) The experimental design to correlate E2F dynamics with commitment into cell cycle entry. Serum-starved cells were released by adding 1% BGS together with EdU and then incubated under time-lapse microscope for E2F1 dynamics measurement. After 44 h incubation, cells were fixed and subjected to EdU staining. (c) EdU labelling after E2F dynamics measurement and cell fixation. Circles mark the nuclei and white arrows indicate cells without EdU signal. Scale bar, 50 μm. (d) Scatter plot based on cell fate (circle, uncommitted; dot, committed) as determined byAmp. Dotted line indicatesAmpth(at which an individual cell has 50% probability to commit into cell cycle). It was determined by using data analysis inf. Solid line indicates the boundary of signal between EdU-positive and -negative cells. 113 cells were analysed. (e) Histogram based on cell fate (red, undivided; green divided) as determined byAmp. 254 cells were analysed by pooling data points from 10, 2 and 1% BGS experimental conditions. (f) Logistic regression curves indicate the probability of cell commitment (dashed line) or division (solid line) as predicted byAmp. The shaded area around each logistic regression curve indicates a 95% confidence interval for 1,000 bootstrapping iterations. Figure 3: Amp as the predictor of commitment and division. ( a ) Linking E2F dynamics to phenotypes in single cells. ( b ) The experimental design to correlate E2F dynamics with commitment into cell cycle entry. Serum-starved cells were released by adding 1% BGS together with EdU and then incubated under time-lapse microscope for E2F1 dynamics measurement. After 44 h incubation, cells were fixed and subjected to EdU staining. ( c ) EdU labelling after E2F dynamics measurement and cell fixation. Circles mark the nuclei and white arrows indicate cells without EdU signal. Scale bar, 50 μm. ( d ) Scatter plot based on cell fate (circle, uncommitted; dot, committed) as determined by Amp . Dotted line indicates Amp th (at which an individual cell has 50% probability to commit into cell cycle). It was determined by using data analysis in f . Solid line indicates the boundary of signal between EdU-positive and -negative cells. 113 cells were analysed. ( e ) Histogram based on cell fate (red, undivided; green divided) as determined by Amp . 254 cells were analysed by pooling data points from 10, 2 and 1% BGS experimental conditions. ( f ) Logistic regression curves indicate the probability of cell commitment (dashed line) or division (solid line) as predicted by Amp . The shaded area around each logistic regression curve indicates a 95% confidence interval for 1,000 bootstrapping iterations. Full size image As we showed that the Amp and k parameters correlate with the commitment into S phase, it stood to reason that they would also predict cell division. To confirm this prediction, we followed cell division over time in single cells and linked it to E2F dynamics. Data points from individual cells stimulated with different serum levels were aggregated and split into two groups depending on whether the cells had divided. A small proportion of cells (<5%) within the undivided group displayed high Amp . These cells were likely within the t 2 interval, and would have been observed to divide if we had kept monitoring them longer ( Supplementary Fig. 3 ). In subsequent analyses, we excluded these cells as we lacked definitive information about their ultimate behaviour. The aggregate data were used to plot the distribution of cells as a function of the values of the corresponding E2F1 dynamic metrics measured in single cells. When plotted against Amp or k , we observed a clear-cut boundary between the group of cells that had divided and the one in which cells had not ( Fig. 3e , Supplementary Fig. 2e ). This distinction became less apparent when the same data were plotted against S and was lost for t 1 or t 2 ( Supplementary Fig. 2f–h ). Next, we performed logistic regression to estimate the probability of cell commitment or division as a function of different metrics [31] . Our results demonstrated that Amp serves as the most accurate predictor, with a confidence value of 95%±1% for commitment (96%±1% for division; Table 1 ). Importantly, we observe an ultrasensitive dependence between the probability of cell commitment/division and the Amp value, reflected in Hill coefficients of >7 for logistic regression curves ( Fig. 3f ). A slight increase of Amp from 2.2 to 2.8 a.u. (12% in the scale of mean Amp in E2F1-activated cells) within the ultra-sensitive region can lead to a 50% relative increase in the proportion of divided cells ( Fig. 3f ). This observed ultrasensitive dependence further defines a threshold value Amp th . If Amp of an individual cell reaches this threshold, it has at least a 50% probability to commit into the cell cycle. Moreover, we observed a similar requirement for Amp in cell-cycle commitment and division in mouse embryo fibroblast NIH3T3 cells, in which the integrated reporter gene was driven by the mouse E2F1 promoter ( Supplementary Fig. 2i–k ). Table 1 Correctness of commitment or division as predicted by different E2F1 dynamics metrics. Full size table Distinct roles of G1 Cyclins and Myc revealed by modelling Considering the predictive power of E2F Amp for individual cells’ commitment to division, we wondered how it would be affected by perturbations on the Rb/E2F network. To this end, we employed an established kinetic model to perform time-course simulations, which can be compared with our experimental observations ( Fig. 1 , Supplementary Tables 1–4 ) [4] , [10] , [32] , [33] . The full model generates E2F transcriptional dynamics that are consistent with our experimental observations ( Supplementary Fig. 4 ). The characteristic E2F pulsatile dynamics are maintained even when each parameter was varied by 100-fold around its base value. We further performed sensitivity analysis of each metric ( Amp , t 2 , k and S ) with respect to changes in 33 parameters in the full model. The analysis indicates that only parameters associated with Myc-dependent E2F autoregulation can lead to dramatic change in Amp ( Supplementary Fig. 5a ). Parameters associated with Myc-dependent E2F autoregulation, Rb-E2F interaction, or CycD and CycE accumulation can significantly affect t 2 , k and S ( Supplementary Fig. 5b–d ). In comparison, parameters associated with the E2F-negative feedback loop have little effect on either Amp , t 2 or k ( Supplementary Fig. 5a–c ). These results suggest that different modules within the full system influence different aspects of E2F dynamics. We next examined the modulation of Amp by perturbations on three main regulators—CycD, CycE and Myc [4] , [11] , [33] . CycD and CycE nodes play a critical role in controlling the function of Rb by phosphorylation, facilitating activation of E2F. They have been suggested as constituting the rate-limiting step in cell cycle entry [1] , [34] . In contrast, Myc has been shown to be critical for modulating the strength of E2F auto-regulation, in addition to contributing to the production of CycD [17] , [18] . We simulated the inhibition of each node by reducing its synthesis rate constant, while maintaining the other model parameters constant. Using our full ordinary differential equation (ODE) model, we ran simulations under a wide range of either CycD or CycE inhibition. Under these conditions, normalized Amp exhibits only a slight decrease ( Fig. 4a,b,d ). In contrast to the robust behaviour of Amp , t 2 shows a significant lengthening as inhibition of either CycD or CycE is increased ( Fig. 4e,f ). Moreover, sensitivity analysis suggests that CycD inhibition has much stronger influence on t 2 extension as compared with CycE inhibition ( Fig. 4h ). This is likely because CycD triggers Rb phosphorylation before CycE further directs additional phosphorylation. We next assessed the consequence of perturbing Myc, as it is known to exert a positive feedback loop on the Rb/E2F network, and to contribute to the bistable property of E2F signalling [17] , [18] . Surprisingly, our simulation analysis indicates that increased inhibition of Myc activity induces a significant decline of normalized Amp ( Fig. 4c,d ). Moreover, t 2 is predicted to moderately increase within the range of inhibition that does not affect the ability of cells to commit ( Fig. 4g,h ). 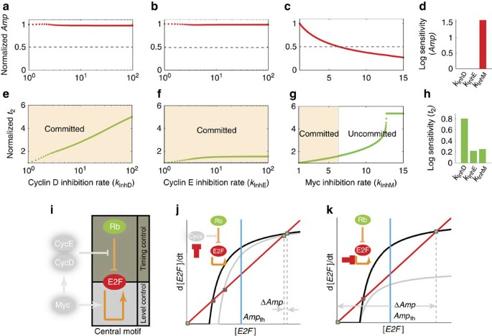Figure 4: Modelling predicts distinct modes of regulation on E2F dynamics by G1 cyclins and Myc. (a–c) NormalizedAmp(to theAmpfor base parameter values) within 120 h under the inhibition of CDK4/6, CDK2 or Myc as function of inhibition rate. Horizontal dashed lines mark that the expected threshold value for normalizedAmpthis 0.5, given that the measuredAmpthis around half of the averageAmpof cells (2.5 versus 5,Fig. 3e). (d) Log sensitivity analysis ofAmpto inhibition rate. (e–g) Normalizedt2to its initial level as a function of inhibition rate under each inhibition case. Yellow shading highlights the region where cells are expected to commit into cell cycle. (h) Log sensitivity analysis oft2to inhibition rate. ForkInhM, log sensitivity was calculated within the committed region. (i) The central motif of Myc/Rb/E2F network includes E2F auto-regulation (module for level control) and its titration by Rb (module for timing control). (j) Steady-state analysis of the central motif under the inhibition of Rb phosphorylation through reduction of cyclin complexes activity. The decrease in Rb phosphorylation rate leads to only a slight reduction (ΔAmp) in steady-state E2F level. Black and grey lines are E2F synthesis curves under low (black) and high (grey) cellular unphosphorylated Rb levels, respectively. Red line indicates the degradation curve. Blue line indicates the thresholdAmpth. Green dots, stable steady states; red dots, unstable steady states. (k) Steady-state analysis of the central motif. Black and grey lines are E2F synthesis curves given high (black) and low (grey) synthesis rate, respectively. Figure 4: Modelling predicts distinct modes of regulation on E2F dynamics by G1 cyclins and Myc. ( a – c ) Normalized Amp (to the Amp for base parameter values) within 120 h under the inhibition of CDK4/6, CDK2 or Myc as function of inhibition rate. Horizontal dashed lines mark that the expected threshold value for normalized Amp th is 0.5, given that the measured Amp th is around half of the average Amp of cells (2.5 versus 5, Fig. 3e ). ( d ) Log sensitivity analysis of Amp to inhibition rate. ( e – g ) Normalized t 2 to its initial level as a function of inhibition rate under each inhibition case. Yellow shading highlights the region where cells are expected to commit into cell cycle. ( h ) Log sensitivity analysis of t 2 to inhibition rate. For k InhM , log sensitivity was calculated within the committed region. ( i ) The central motif of Myc/Rb/E2F network includes E2F auto-regulation (module for level control) and its titration by Rb (module for timing control). ( j ) Steady-state analysis of the central motif under the inhibition of Rb phosphorylation through reduction of cyclin complexes activity. The decrease in Rb phosphorylation rate leads to only a slight reduction (Δ Amp ) in steady-state E2F level. Black and grey lines are E2F synthesis curves under low (black) and high (grey) cellular unphosphorylated Rb levels, respectively. Red line indicates the degradation curve. Blue line indicates the threshold Amp th . Green dots, stable steady states; red dots, unstable steady states. ( k ) Steady-state analysis of the central motif. Black and grey lines are E2F synthesis curves given high (black) and low (grey) synthesis rate, respectively. Full size image As the G1 cyclin and Myc are both positive regulators of E2F, their qualitatively different impact on E2F Amp appears counter intuitive. Nevertheless, close inspection indicates that this is an intrinsic dynamic property of the underlying network. To illustrate the control logic, we simplified the network to a motif comprising an E2F-positive feedback and a negative regulation through Rb sequestration ( Fig. 4i ). Other regulatory inputs impinge on this motif by affecting the positive feedback loop strength or affecting Rb phosphorylation. This motif can be described by a single equation (1): where [ E2F ] represents E2F concentration, [ Rb ] the concentration of active Rb (unphosphorylated) that can bind to and titrate E2F, [ E2F ] e the concentration of free E2F, k syn the E2F synthesis rate constant, K the half-maximal constant for E2F auto-regulation and d the degradation rate constant. This equation describes the dynamics of the motif in the limiting case of extremely tight binding between Rb and E2F. As illustrated by our steady-state analysis, inhibition of Myc drastically reduces the E2F amplitude by decreasing E2F synthesis rate, suggesting that Myc is largely responsible for setting maximum levels of E2F ( Fig. 4k ). In contrast, inhibition of CycD or CycE decreases the phosphorylation rate of Rb, which acts as a ‘sink’ against the initial E2F activation. Despite the drastic slowdown in phosphorylation, and as long as Rb gets completely phosphorylated by Cyclin/CDK complexes, E2F will reach its maximum level set by Myc ( Fig. 4j ). As a result, inhibition of the cyclin nodes primarily modulates the time it takes to overcome the Rb-sink but has little impact on the eventual E2F amplitude. Control of timing but not commitment by G1 Cyclin/CDKs To experimentally monitor the behaviour of the network after CycD/E inhibition, we used the CDK4/6- and CDK2-specific inhibitors—PD0332991 and CVT-313—in a wide range of concentrations [35] , [36] , [37] , [38] . We confirmed the inhibitory effect at each concentration by monitoring phosphorylation of Rb at various Ser or Thr residues ( Supplementary Fig. 6a ). To exclude the possibility of an off-target effect from CDK2 inhibition, we generated short hairpin RNAs (shRNAs) to knockdown endogenous CDK2 level ( Supplementary Fig. 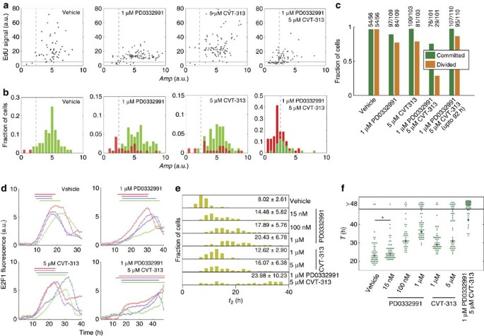Figure 5: Control of timing in cell-cycle progression but not commitment decision by G1 Cyclin/CDK complexes. (a) Scatter plot based on commitment as determined byAmpunder inhibition of CDKs (PD0332991 for CDK4/6 and CVT-313 for CDK2). Committed cells were measured by EdU labelling after 48 h incubation, and divided cells were counted 48 h after addition of 10% BGS. (b) Histogram based on cell division as determined byAmpunder inhibition of CDKs (48 h observation). (c) Proportion of committed/divided cells under different inhibitions of CDKs during a 48- and 92-h (the latter only for the combined inhibition) observation window. The exact number of total cells followed and that of cells committed/divided are indicated on top of each error bar. (d) Four representative E2F1 dynamics trajectories under the same conditions asa. Each colour bar on top indicates the length oft2of its corresponding trajectory. (e) Distribution oft2of individual cells in mock, CDK4/6-, CDK2- and combinational inhibited samples. Mean±s.d. is shown on top right of each panel. 54 (Vehicle), 106 (15 nM PD0332991), 102 (100 nM PD0332991), 109 (1 μM PD0332991), 94 (1 μM CVT313), 105 (5 μM CVT313) and 101 (1 μM PD0332991 and 5 μM CVT313) cells were analysed for each condition, respectively. (f) Plot of the first cell cycle length (T) under the condition as ine. Every dot represents a single cell. Black cross indicates the median ofTamong the cells divided within 48 h. *P=0.01855, Wilcoxon one-side test. For all testing results,P<0.005 unless marked. 6e , Supplementary Table 5 ). Single-cell analysis of E2F1 dynamics after serum stimulation was combined with EdU incorporation or visual inspection of cell division in the presence of the CDK4- and CDK2-specific inhibitors or CDK2 shRNA. Consistent with our modelling analysis, inhibition of CycD or CycE complexes had no effect on the distribution of Amp (<5% of cells found in the OFF mode; Fig. 5a,b , Supplementary Fig. 6b ). Inhibition of both complexes moderately increased the proportion of cells showing a low-mode Amp (~25% of cells in the OFF mode) given a 48-h observation window ( Fig. 5a,b , Supplementary Fig. 6b ). When cells were monitored for cell division, we observed that inhibition of CycD or of CycE complexes (or both) led to a decrease in the fraction of cells that completed division during the time window of our assay ( Fig. 5c ). However, it had little effect on the fraction of cells that incorporated EdU (and presumably had committed to the cell cycle; Fig. 5c , Supplementary Fig. 6f ). Figure 5: Control of timing in cell-cycle progression but not commitment decision by G1 Cyclin/CDK complexes. ( a ) Scatter plot based on commitment as determined by Amp under inhibition of CDKs (PD0332991 for CDK4/6 and CVT-313 for CDK2). Committed cells were measured by EdU labelling after 48 h incubation, and divided cells were counted 48 h after addition of 10% BGS. ( b ) Histogram based on cell division as determined by Amp under inhibition of CDKs (48 h observation). ( c ) Proportion of committed/divided cells under different inhibitions of CDKs during a 48- and 92-h (the latter only for the combined inhibition) observation window. The exact number of total cells followed and that of cells committed/divided are indicated on top of each error bar. ( d ) Four representative E2F1 dynamics trajectories under the same conditions as a . Each colour bar on top indicates the length of t 2 of its corresponding trajectory. ( e ) Distribution of t 2 of individual cells in mock, CDK4/6-, CDK2- and combinational inhibited samples. Mean±s.d. is shown on top right of each panel. 54 (Vehicle), 106 (15 nM PD0332991), 102 (100 nM PD0332991), 109 (1 μM PD0332991), 94 (1 μM CVT313), 105 (5 μM CVT313) and 101 (1 μM PD0332991 and 5 μM CVT313) cells were analysed for each condition, respectively. ( f ) Plot of the first cell cycle length ( T ) under the condition as in e . Every dot represents a single cell. Black cross indicates the median of T among the cells divided within 48 h. * P =0.01855, Wilcoxon one-side test. For all testing results, P <0.005 unless marked. Full size image In contrast, and consistent with our simulation results, inhibition of CycD, CycE or both led to significant increases in t 2 and its variance ( Fig. 5d,e , Supplementary Fig. 6g ). The prolonged t 2 results in a significant extension of the entire cell cycle length ( Fig. 5f , Supplementary Fig. 6h ). As t 1 and t 3 show moderate changes under inhibition of CycD/E ( Supplementary Fig. 6c and d ), the increase in t 2 is the primary contributor to cell cycle elongation. For this reason, the observed reduction in the proportion of cells that undergo cell division under dual inhibition is likely an overestimation. Indeed, we found a significant increase in the proportion of divided cells and the recovery of Amp distribution in the case of combined inhibition if we extended the time of observation to 92 h ( Fig. 5c , Supplementary Fig. 6b ). Our experimental data therefore validate the predictions from the model and suggest that cells under CycD/E inhibition can commit to cell cycle entry but progress more slowly on the way to cell division. Control of commitment into cell cycle entry by Myc To experimentally test the functional consequences induced by Myc inhibition, quiescent cells were stimulated with full serum in the presence of EdU and of different concentrations of either Myc-specific inhibitor 10058-F4 (which efficiently interferes with Myc/Max hetero-dimerization) or the bromodomain inhibitor (+)-JQ1 (which substantially suppresses c-Myc transcription) [39] , [40] , [41] , [42] , [43] , [44] ( Supplementary Fig. 7a ). Consistent with our modelling analysis, single-cell analysis indicates that Myc inhibition dramatically prevents Amp to switch from an OFF mode to an ON mode, resulting in a sharp decrease in the proportion of both committed and divided cells ( Fig. 6c , Supplementary Fig. 7b ). Fitting the curves to a Hill function yielded a sharp sigmoid pattern for both division and commitment ( Fig. 6c , Supplementary Fig. 7b ). Moreover, we note a bimodal response at an intermediate inhibitor level (90 μM for 10058-F4 and 0.8 μM for (+)-JQ1; Fig. 6a,b , Supplementary Fig. 7c and d ), which is around the half-inhibition threshold. At this dose, part of the cells was able to commit and they exhibited a strong E2F response ( Fig. 6d ). In contrast, the other cells remained in quiescence and they exhibited weak E2F responses ( Fig. 6d ). We also performed shRNA knockdown of endogenous c-Myc level to rule out the potential for a non-specific effect of the inhibitors ( Supplementary Fig. 7e , Supplementary Table 5 ). A large proportion of the cells remained in the OFF mode after serum stimulation, fully supporting our findings obtained with two independent small-molecule inhibitors of Myc ( Supplementary Fig. 7f ). All these results are consistent with the bistable nature of E2F activation in response to upstream signals and suggest a critical role for Myc in this regulation [4] . Importantly, they further underscore the predictable power of the parameter Amp in E2F dynamics for cell cycle commitment. 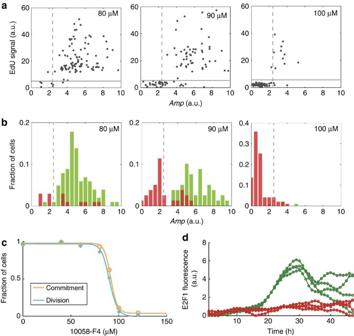Figure 6: Control of commitment into cell cycle entry by Myc. (a) Scatter plot of commitment as determined byAmpunder different c-Myc inhibitor (10058-F4) concentrations (80, 90 and 100 μM). 101, 100 and 93 cells were analysed for each condition. (b) Histogram of cell division as determined byAmpunder the conditions ina. (c) Dose–response curves (fitted to data points as Hill functions) indicate the proportion of divided/committed cells under different c-Myc inhibitor concentrations. (d) Representative E2F1 dynamics trajectories (green for committed cells; red for uncommitted cells) at 90 μM 10058-F4 inhibitor concentration. Figure 6: Control of commitment into cell cycle entry by Myc. ( a ) Scatter plot of commitment as determined by Amp under different c-Myc inhibitor (10058-F4) concentrations (80, 90 and 100 μM). 101, 100 and 93 cells were analysed for each condition. ( b ) Histogram of cell division as determined by Amp under the conditions in a . ( c ) Dose–response curves (fitted to data points as Hill functions) indicate the proportion of divided/committed cells under different c-Myc inhibitor concentrations. ( d ) Representative E2F1 dynamics trajectories (green for committed cells; red for uncommitted cells) at 90 μM 10058-F4 inhibitor concentration. Full size image Quantitative analysis of real-time dynamics of E2F1 transcription in single mammalian cells has allowed us to define the metrics that accurately predict cell commitment and proliferation. We find that the values of Amp and t 2 respond to two intimately linked but differentially controlled modes of regulation by the Myc/Rb/E2F network. Amp is critically dependent on Myc activity, whereas t 2 is highly sensitive to the activity of G1 cyclin complexes. Amp serves as the single most reliable predictor of cell cycle commitment in single cells. In particular, we show an ultrasensitive dependence on Amp for the probability of each individual cell to commit into the cell cycle. Importantly, this predictive power is probabilistic in nature. If Amp is at Amp th (2.5), a cell has a 50% chance to commit. However, a slight increase in Amp (from 2.2 to 2.8) greatly boosts the probability (from 25 to 75%). In this case, because of the stochastic nature of single-cell behaviour, there is still a small probability by which a cell can stay in quiescence. In the temporal scale, transition across the Amp th defines a critical time point after which a cell becomes likely to commit into division. This time point is reminiscent of the classical restriction point [34] , [45] , but has the advantage that it can be precisely determined in single cells. Remarkably, Amp has remained a reliable predictor of cell cycle commitment even under drastic perturbations of the Myc/Rb/E2F network in REF52 and NIH3T3 fibroblasts. As this network is highly conserved among different tissues and species [5] , it will be interesting to test the generality of this principle among different cell types, including normal and cancerous cells. On the other hand, t 2 seems to account for the main variability for cell cycle duration, as its variation correlates with that of the cell cycle length. At the temporal scale, t 2 covers the late G1 phase and most (if not all) of S phase. This time window is most variable during the cell cycle, perhaps allowing cells to optimize conditions for the completion of the cell cycle in response to internal stress signals such as DNA damage response [46] . Although the role of the Rb/E2F pathway in regulating the cell cycle has been well documented, the precise contribution of how its core constituents mediate temporal steps in its execution has not been fully established. Our single-cell analysis of E2F activation dynamics has generated new mechanistic insights into this issue. First, we find that Myc is critical for cell cycle entry. Myc has long been recognized as a potent proto-oncogene, and its effect on cell proliferation was largely attributed to its regulation of G1 cyclins expression and CDK activities [16] , [47] , [48] . However, our results show that Myc’s contribution is primarily due to its direct modulation of the E2F Amp . Our findings therefore challenge the general view that G1 cyclins are predominantly responsible for controlling the commitment to cell cycle entry. Instead, our results show that the primary role of G1 cyclins is to tune the timing and duration of the cell cycle. This conclusion is consistent with observations in knockout mouse models where G1 cyclins and CDKs are largely dispensable for cell cycle entry, although they affect efficacy or timing of commitment [49] , [50] , [51] , [52] , [53] . Taken together, our results reveal that the Myc/Rb/E2F network coordinates two independent control modes of cell cycle progression: the decision of ‘whether’ by Myc and that of ‘when’ by G1 cyclins. These two control modes may also be targeted to regulate cell cycle exit. For instance, reduction of Myc levels and activity would lead to a quick exit from the cell cycle, as is required for contact inhibition or terminal differentiation [14] , [54] . Furthermore, potent inhibition of G1 cyclins would likely trap cells in an infinitely long and futile cell cycle, resulting in cellular senescence. Yao et al. [4] have established the relationship between bistable E2F activation and the crossing of the restriction point using flow-cytometry measurements. In contrast, use of fluorescence microscopy enabled us to measure E2F temporal dynamics in single cells, and to correlate this information with single-cell decisions. Our approach revealed a clear distinction in the roles that Myc and G1 cyclins have on the control of E2F activation. Our results reveal an unappreciated and critical requirement for Myc-dependent E2F autoregulation that controls the cell-cycle commitment decision of fibroblasts released from G0 after serum stimulation. Using a CDK2 activity reporter, Spencer et al. [55] recently reported that the proliferation-to-quiescence decision in continuously growing cells is controlled by a bifurcation in CDK2 activity after mitotic exit. They also showed that the bifurcation is regulated by the CDK inhibitor p21 and mitogen signals. It is interesting to note that the stability of Myc is tightly regulated by mitogen signals through MAPK and Akt pathways [56] , [57] . Moreover, p21 can function as a repressor of Myc transcription or directly interfere with Myc transcriptional activity by blocking Myc/Max complex formation [58] , [59] . Given our finding that Myc is the driver of cell cycle commitment, Myc activity may also influence the control of proliferation-to-quiescence decision by p21 and mitogen signals. Therefore, it will be interesting to combine the E2F and CDK2 reporter systems together to better understand the temporal and mutual (if any) relationship in the dynamics of these two factors and to investigate how Myc, CDK2, p21 and the mitogen signals combine to regulate the normal cell cycle. Last, the measurement of single-cell E2F dynamics provides a quantitative and sophisticated framework for understanding the control logic of cell cycle entry. Clear delineation of the precise function of each effector in the Myc/Rb/E2F network implicated in cell cycle control has implications for developing effective strategies for cancer therapy. E2F1 transcriptional reporter system A DNA fragment encoding d4Venus (destabilized Venus with ~4 h half-life) was cut from pd4Venus-N1 and fused with four repeats of SV40 nuclear localization sequence (NLS) at its N-terminus to generate the 4NLS-d4Venus-expressing cassette [60] . This cassette was then sub-cloned after the human E2F1 promoter (−784 to +32) into a pQCXIP vector (Clontech) to construct the pQCXIP-hE2F1p::4NLS-d4Venus reporter plasmid [17] . The derived construct was transfected into an ecotropic packaging cell line, Plat-E [61] . Forty-eight hours after transfection, the culture medium containing retrovirus particles was filtered and applied to REF52 cells. A clonal pool genetically integrated with the reporter system was selected after cells were cultured in medium containing puromycin (2 μg ml −1 ) for approximately 10 days. Single clones (REF52-hE2F1p::4NLS-d4Venus) were then picked up from the clonal pool by dilution. The developed hE2F1p::4NLS-d4Venus reporter system leads to two significant improvements appropriate for single-cell analysis. On one hand, the incorporation of four NLSs in the protein drives its localization into the nucleus, thereby increasing the intensity of the fluorescent signal. On the other hand, it facilitates segmentation and signal extraction in individual cells, as nuclei in different cells are well separated. Based on a similar strategy, a mouse E2F1 promoter (−1,165 to +123) was amplified from mouse genomic DNA as a substitute for human E2F1 promoter to derive the construct pQCXIP-mE2F1p::4NLS-d4Venus, which was later introduced into mouse embryonic fibroblast NIH3T3 cells to derive the NIH3T3-mE2F1p::4NLS-d4Venus reporter cells. Cell culture REF52 (an immortal line of postcrisis Fischer rat embryo cells) [4] , [62] , [63] and NIH3T3 mouse fibroblasts (CRL-1658, ATCC) were routinely grown in Minimum Essential Medium Alpha Medium (Gibco/Invitrogen) supplemented with 10% bovine growth medium (BGS, Hyclone/Thermo Scientific). For the preparation of E2F dynamics measurement by using time-lapse microscopy, cells were first trypsinized, resuspended at a density of 1 × 10 5 per ml and then seeded in μ-Slide I (tissue culture treated, ibidi) channel slides by adding 1 ml volume of the cell suspension. After overnight culturing, cells were synchronized in quiescence by shifting into Minimum Essential Medium Alpha medium with 0.02% BGS (starvation medium) for 36 h. For perturbation experiments, PD0332991 (CDK4/6 inhibitor, ChemieTek), CVT-313 (CDK2 inhibitor, Enzo Life Science), 10058-F4 (c-Myc inhibitor, Sigma Aldrich) and (+)-JQ1 (bromodomain and extra terminal domain inhibitor, Cayman Chemical) were added into cells immediately after cells were released from serum starvation (by adding 10% BGS) in either single or combined way. For 92 h perturbation experiment with both PD0332991 and CVT-313, cells were growing with replaced fresh medium with fresh inhibitors after the initial 48 h. Live cell imaging For time-lapse microscopy, quiescent cells growing in μ-Slide I slides were released from starvation by shifting to serum containing medium and placed under Leica DMI 6000 B inverted fluorescence microscope (Leica). Images were taken using Leica N PLAN L 20 × 0.4 objective lens with phase contrast or a Semrock BrightLine YFP filter set (500/542 nm, excitation/emission) and Hamamatsu ORCA AG digital camera (Hamamatsu) with uniform parameter setting: binning=4, offset=0, gain=255 and exposure time=0.01 s (phase channel) or 0.15 s (YFP channel). The microscope was enclosed with an environmental chamber with 37 °C temperature, atmosphere (5% CO 2 ) and humidity. Images were acquired every 30 or 60 min for 24–48 h. Time-series image acquisition was controlled by SimplePCI6 Software (Hamamatsu). EdU staining and imaging EdU staining was performed after E2F dynamics measurement in ibidi μ-Slide I slides by using Click-iT EdU Imaging Kits (Invitrogen) with Alexa Fluro 594 azide according the manufacturer’s instructions. The only modification of the protocol was to wash cells with PBS with 0.2% Tween three times after all the staining steps. Images were taken using Leica N PLAN L 20 × 0.4 objective lens with phase contrast or a Semrock BrightLine Texas Red filter set (562/624 nm, excitation/emission) and Hamamatsu ORCA AG digital camera with uniform parameter setting: binning=4, offset=0, gain=255 and exposure time=0.01 s (phase channel) or 0.8 s (Red channel). Western blot analysis Antibodies against E2F1 (1:1,000, Cell Signaling), phosphorylated Rb Ser 780 (C-15, 1:1,000, Santa Cruz), phosphorylated Rb Thr 821/826 (sc-16669-R, 1:1,000, Santa Cruz), GFP (XP Rabbit mAb, 1:1,000, Cell Signaling), c-Myc ((D84C12) XP Rabbit mAb, 1:1,000, Cell Signaling), CDK2 (78B2 Rabbit mAb, 1:1,000, Cell Signaling) and Actin (C-2, 1:1,000; Santa Cruz) were selected for the quantification of protein expression at the population level. REF52-E2F1p::4NLS-d4Venus cells were harvested and protein extract was obtained by lysis at different time points after release from quiescence. Total protein amount was quantified with the BCA assay (Pierce). Equal protein amounts were separated by 4–20% Mini PROTEAN TGX gradient gels (Bio-Rad) and transferred to polyvinylidene membranes by electro-blotting. Membranes were then blocked with 5% nonfat dried milk, incubated overnight at 4 °C with primary antibody, washed in TBS with 0.2% Tween, and incubated again with secondary antibody coupled to peroxidase. Protein levels were detected by using LumiGLO Peroxidase Chemiluminescent Substrate Kit (Cell Signaling) after additional washing steps. All the photos of full blots are displayed in Supplementary Fig. 9 . Quantitative reverse transcription–PCR analysis RNA extracts were prepared from REF52-hE2F1p::4NLS-d4Venus reporter cells using the RNeasy Protect Cell Mini Kit (Qiagen) according to the manufacturer’s protocol. E2F1 RNA expression was interrogated by real-time PCR using the Power SYBR Green RNA-to-C T 1-step Kit (Applied Biosystems). Gene-specific primers used: 5′-TTGACCCCTCTGGATTTCTG-3′ and 5′-CCCTTTGGTCTGCTCAATGT-3′ for rat E2F1; 5′-GTCGTACCACTGGCATTGTG-3′ and 5′-CTCTCAGCTGTGGTGGTGAA-3′ for rat β-actin. RNA interference shRNAs for targeting CDK2 or c-Myc were generated by cloning shRNA sequences ( Supplementary Table 5 ) into Tet-pLKO-2A-mCherry vector [64] . Lentiviral packaging reactions were performed in the 293T cell line in the presence of packaging plasmids psPAX and pMD2.G using Lipofectamine Transfection Reagent (Invitrogen). Viral supernatants were collected 48 h after transfection, filtered through disposable 0.45 μm acrodisc syringe filters (Pall Corporation). For infection, cells were plated in 10 cm tissue culture dishes and allowed to achieve 20–30% confluence before adding viral supernatant in the presence of 7 μg ml −1 polybrene for 12 h (EMD Millipore). Cells were collected and sorted by flow cytometry for 5% of the population with highest mCherry signals. Sorted cells were grown up and induced to express shRNA at different concentration of doxycycline (Sigma-Aldrich) for 48 h. After induction, cells were lysed and knockdown efficiency was determined by western blot analysis. Meanwhile, sorted cells with confirmed knockdown effect were subjected to the measurement of E2F dynamics in the presence of doxycycline at different doses. Image analysis The time-lapse microscopy resulted in two series of raw images of the cells in 30 or 60-min increments for 24–48 h, one each for the phase channel and the YFP channel. E2F signals were extracted from these images using ImageJ (NIH) software. The first time-point of each series of images was loaded side-by-side into the software. Using the ROI Manager Tool, a circular selective marker with a fixed area was placed around each cell nucleus in the phase channel image. The location of each marker was then copied to the YFP channel image and the integrated grey value of the selected pixels was measured. In the case of cell division, the selective marker was applied to one of the daughter cells. This value was normalized to the background by subtracting the integrated grey value of the same area of pixels in an empty part of the image. This process of measuring normalized grey value of the nuclei was repeated for each time point by adjusting the location of the selective marker to account for the movement of cells, thus giving a time-series measurement of the fluorescence reporter on the E2F sequence. Throughout this process, data from cells that left the field of view at any time were discarded; and the time of cell division was also noted. The similar approach was applied to quantify the fluorescence signal from EdU staining. Analysis of E2F dynamics trajectories Time-series E2F dynamics trajectories were analysed in Matlab (MathWorks) to determine various E2F parameters, for example, time delay, amplitude and so on. We developed a smoothing algorithm based on the recognition to remove the large fluorescence spike that occurs during mitosis, possibly as a result of either the increased concentration of endogenous E2F that accompanies cell mass shrinkage or the change from a ‘flat’ to a ‘globular’ cell shape that immediately precedes division. The processed trajectories without spikes were then smoothened by using a three-window Gaussian averaging algorithm. Each smoothed and processed trajectory was then fit to the following two-phase regression model (equation (2), Supplementary Fig. 8 ) to automatically derive optimal values for t 1 and t 2 (ref. 65 ): Thus, the problem equals to search for arg { t 1 , t 2 } that gives min { ∑ 0 ≤ t ≤ t 2 [ y E2F ( t ) − y ( t )] 2 }. Relevant parameters represent: t 1 : initial delay t 2 : activation time y 0 : E2F basal level (the average of fluorescence values of the initial four time points) y max : E2F peak level (maximum fluorescence value of each trajectory) y E2F ( t ): E2F signal in dynamic trajectory at the moment t . Modelling and simulation analysis A modified version of a previously developed ODE model of Myc/Rb/E2F network was applied for simulation analysis [4] , [11] . Compared with models applied in previous analysis, we neglected the hypothetical feed-forward loop from Myc to E2F and microRNA-mediated negative feedback loops, rendering the model more concise but completely maintain essential regulatory characteristics. However, we include a representative factor R , which represents regulators in E2F-related negative feedback loops, such as Cyclin A and Skp2 ( Fig. 1 ) [19] , [20] , [66] . The introduction of R does not influence stead-state analysis, but shapes the curves with slight decrease after Amp reaching the maximum level, which is consistent with experimental observation. Given the fact that Myc and Cyclin D levels usually rise 6–8 h after serum addition during cell cycle entry [67] , we reasoned that the initial delay ( t 1 ) is mainly due to the delayed activation of these upstream factors. Therefore, we performed simulation with an initial constraint that Myc and Cyclin D are forced to be zero until the simulation precedes to 8-h time point at the temporal scale. Simulations based on these assumptions were able to generate E2F dynamics trajectories including a significant length of t 1 ( Supplementary Fig. 4 ). On the other hand, we noted the fact that a time lag exists between Cyclin E activation and that of Cyclin A [68] , [69] . Moreover, population dynamics of Skp2 show a peak after that of E2F1 (ref. 20 ). Therefore, we reasoned that the activation of negative feedback loop through R is a delayed event after E2Fp increases. We introduced a time lag between these two events by setting a threshold for E2Fp (0.4 μM), above which E2F starts to transcribe R . The introduction of this delayed negative feedback loop was able to generate a slight decrease in E2Fm dynamics after it reaches the peak level, consistent with our experimental observations ( Fig. 2c,d ). To mimic the perturbation of Cyclin D/E or Myc node, we multiplied the degradation term with a coefficient ( k Inh , inhibition rate) as shown in the following equation (3): Through varying the inhibition rate k Inh within a wide range (1- to 100-fold), we performed simulations and derived a series of E2F temporal trajectories. The normalized peak values of E2F (corresponding to Amp ) for each trajectory were calculated and plotted against the inhibitor concentration ( Fig. 4a–c ). t 2 was calculated from each trajectory by using the similar method as described above and plotted as Fig. 4e–g . Log sensitivity analysis Log sensitivity of the four metrics to each parameter was calculated by the following equation (4): How to cite this article: Dong, P. et al. Division of labour between Myc and G1 cyclins in cell cycle commitment and pace control. Nat. Commun. 5:4750 doi: 10.1038/ncomms5750 (2014).